Structural insights into the role of the Smoothened cysteine-rich domain in Hedgehog signalling Smoothened (Smo) is a member of the Frizzled (FzD) class of G-protein-coupled receptors (GPCRs), and functions as the key transducer in the Hedgehog (Hh) signalling pathway. Smo has an extracellular cysteine-rich domain (CRD), indispensable for its function and downstream Hh signalling. Despite its essential role, the functional contribution of the CRD to Smo signalling has not been clearly elucidated. However, given that the FzD CRD binds to the endogenous Wnt ligand, it has been proposed that the Smo CRD may bind its own endogenous ligand. Here we present the NMR solution structure of the Drosophila Smo CRD, and describe interactions between the glucocorticoid budesonide (Bud) and the Smo CRDs from both Drosophila and human. Our results highlight a function of the Smo CRD, demonstrating its role in binding to small-molecule modulators. Smoothened (Smo), a member of the Frizzled (FzD) class of G-protein-coupled receptors (GPCRs) is an integral member of the Hedgehog (Hh) signal transduction cascade, first identified through genetic analysis in fruit fly Drosophila melanogaster [1] , [2] , [3] , [4] . The Hh pathway plays an important role during embryogenesis controlling cell maturation, differentiation and proliferation [5] , [6] . Disruption of Hh signalling during development leads to a plethora of developmental anomalies [7] , [8] . Conversely, ectopic Hh signalling during adult life contributes to tumour development and progression, particularly in cancers including medulloblastoma, basal cell carcinoma and rhabdomyosarcoma [9] . Consequently, the pathway is an important therapeutic target in oncology and regenerative medicine. The Hh signal is transduced in a sequential manner that is initiated by the endogenous ligand Indian, Sonic or Desert Hh binding to the 12 transmembrane protein Patched (Ptc) to attenuate its housekeeping inhibition of Smo [10] , [11] , [12] , [13] . Smo then translocates to the cell membrane in Drosophila, or the primary cilium in vertebrates, and induces downstream signalling to the Gli/Cubitus interruptus transcription factors [5] , [13] . The crystal structure of the seven transmembrane (7TM) domain of human Smo was recently elucidated [14] . This structure revealed the canonical GPCR 7TM helical fold along with the conformation of the extracellular loop (ECL) and an extracellular linker domain (ECLD), both of which are stabilized by disulphide bonds between the conserved cysteine residues [14] , [15] . However, the major portion of the Smo extracellular domain (ECD) is the cysteine-rich domain (CRD), which was not included in the crystal structure of the Smo receptor [14] . The CRDs of FzD family GPCRs possess modest homology. Nevertheless, the cysteines in this domain are highly conserved [16] , [17] . While the CRD of FzD plays an essential role in Wnt ligand binding and receptor dimerization [16] , [18] the role of the Smo CRD is not clear, although it has been shown that the Smo CRD is indispensable for Hh signalling in both Drosophila and vertebrates [19] , [20] . Drosophila and vertebrate Smo lacking the CRD fail to cycle to the plasma membrane or primary cilium to induce maximum signalling [19] , [20] . Furthermore, in Drosophila CRD deletion mutants fail to dimerize, suggesting that the CRD may govern Smo dimerization [21] . On the basis of its functional importance, and the observation that the related FzD CRD binds to Wnt, it has been speculated that the Smo CRD may facilitate binding of an as yet unidentified, endogenous small molecule that modulates Smo signalling activity in the presence of Hh [19] . Recent studies have identified two major groups of small molecules capable of modulating Smo signalling activity: hydroxyl-sterols and glucocorticoids, both of which modulate Hh signalling through governing subcellular localization and activity of Smo [22] , [23] . Twenty hydroxycholesterol (20-OHC) and budesonide (Bud) have been reported to bind to a Smo domain distinct from the orthosteric site present in the transmembrane core, previously demonstrated to bind the inhibitory small-molecule cyclopamine [22] , [23] , [24] . Recent reports also indicate that 20-OHC binds the vertebrate Smo CRD [25] , [26] . Therefore, we hypothesized that the CRD of Smo may act as an allosteric binding site for Bud and additional small-molecule Smo modulators. To test this hypothesis, and to gain more insight into the functional significance of the Smo CRD, we performed structure–function studies. Here we present the first solution structure of the Drosophila Smo CRD. We demonstrate that the CRD possesses a conserved pocket that contributes to the binding and allosteric regulation by the small-molecule Bud. The Smo CRD is essential for Hh signalling The Smo CRD is essential for regulating its subcellular localization and signalling [19] , [20] , [21] . The cysteines in this domain are conserved from Drosophila through vertebrates ( Fig. 1 ). Despite this essential role, the functional contribution of the CRD to Smo regulation has remained unclear. To gain functional insight into the role of the CRD, we generated a mutant lacking this domain (ΔCRD; V85-K202), and tested its ability to rescue Hh-dependent reporter gene induction following knockdown of endogenous smo in cultured Clone 8 (Cl8) cells [27] . Consistent with previous in vivo studies, we found that deletion of this domain ablates Smo signalling capacity in vitro ( Fig. 2 ). To better dissect this essential functional domain, we studied the structure of the Smo CRD using NMR methods. 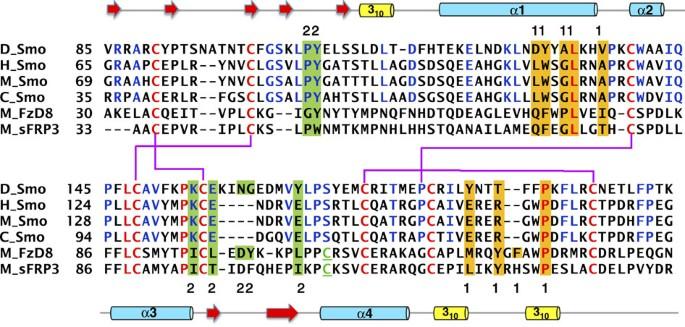Figure 1: Sequence alignment of the Smo CRD. Primary sequence alignment of theDrosophila(D), human (H), mouse (M) and chicken (C) Smo CRD with that of mouse FzD8 CRD and mouse-secreted FzD Related Protein 3 (sFRP3). The residues conserved in Smo and FzD CRD are shown in red, whereas the residues conserved only in the Smo CRD are shown in blue. The cysteine in FzD not conserved in Smo is underlined and shown in green. The disulphide bond pattern for the Smo CRD is shown in thick purple lines. The secondary structure elements are shown above and below the primary sequence. The residues highlighted in orange indicate the ‘site 1’ residues of mouse FzD8 that interact with the palmitate modification on the ligand Wnt. The residues highlighted in green indicate the ‘site 2’ on mouse FzD8 that interact with the amino-acid side chains on the opposite side of Wnt. The sequence alignment was generated using ClustalW2. Figure 1: Sequence alignment of the Smo CRD. Primary sequence alignment of the Drosophila (D), human (H), mouse (M) and chicken (C) Smo CRD with that of mouse FzD8 CRD and mouse-secreted FzD Related Protein 3 (sFRP3). The residues conserved in Smo and FzD CRD are shown in red, whereas the residues conserved only in the Smo CRD are shown in blue. The cysteine in FzD not conserved in Smo is underlined and shown in green. The disulphide bond pattern for the Smo CRD is shown in thick purple lines. The secondary structure elements are shown above and below the primary sequence. The residues highlighted in orange indicate the ‘site 1’ residues of mouse FzD8 that interact with the palmitate modification on the ligand Wnt. The residues highlighted in green indicate the ‘site 2’ on mouse FzD8 that interact with the amino-acid side chains on the opposite side of Wnt. The sequence alignment was generated using ClustalW2. 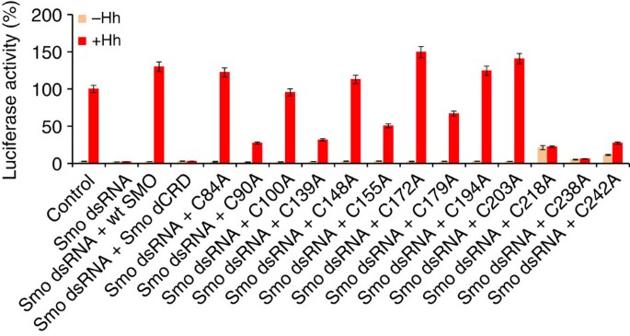Figure 2: Identification of cysteines essential for Smo signalling. CRD residues C90, C139, C155, C179 and the Smo ECLD residues C218, C238 and C242 are required for proper Hh reporter gene induction. Mutation of C84, 100,148,172,194,203 to alanine did not compromise the ability of Smo protein to induce the Hh reporter gene activity, and behaved similar to the wild-type protein. Percent activity for each of the experimental assays is shown relative to control. The control level of Hh-induced, ptcΔ136-luciferase activity for control dsRNA was set to 100%. For all conditions, luciferase activity is normalized topAc-renillacontrol. Experiments were performed a minimum of two times in duplicate or triplicate and all data were pooled. Error bars indicate s.e.m. Full size image Figure 2: Identification of cysteines essential for Smo signalling. CRD residues C90, C139, C155, C179 and the Smo ECLD residues C218, C238 and C242 are required for proper Hh reporter gene induction. Mutation of C84, 100,148,172,194,203 to alanine did not compromise the ability of Smo protein to induce the Hh reporter gene activity, and behaved similar to the wild-type protein. Percent activity for each of the experimental assays is shown relative to control. The control level of Hh-induced, ptcΔ136-luciferase activity for control dsRNA was set to 100%. For all conditions, luciferase activity is normalized to pAc-renilla control. Experiments were performed a minimum of two times in duplicate or triplicate and all data were pooled. Error bars indicate s.e.m. Full size image Solution structure of the Smo CRD A recombinant Drosophila Smo CRD (V85-K202) was expressed and purified using the Escherichia coli expression system. For the purpose of NMR studies, 15 N- and 13 C-labelled protein was prepared in 10 mM deuterated acetic acid buffer and 10% D 2 O (volume/volume) at pH 5. Resonance assignments were performed using the standard triple resonance strategy for 13 C-, 15 N-labelled proteins [28] . In the two-dimensional (2D) 1 H– 15 N heteronuclear single quantum coherence (HSQC) spectra, all the amide resonances of the 118 residues of the CRD could be observed except D116. D116 is in the loop region preceding the first helix and hence could be undergoing motions in the intermediate timescale resulting in peak broadening for the backbone amide; nevertheless, all the side-chain resonances of this residue were observed. Using the structural information obtained from the NMR studies, 100 structures were calculated and the 20 structures with the lowest energy are represented as an ensemble ( Fig. 3a ). The statistical details for the NMR structure calculation are given in Table 1 . The structure has no distance violation >0.03 Å and no angle violations >1 o . The structure with the lowest energy is used to describe the secondary structure elements ( Fig. 3b ). The tertiary fold of the Smo CRD is very similar to that of the FzD CRD [16] , [18] ( Fig. 3c , cyan compared with red). 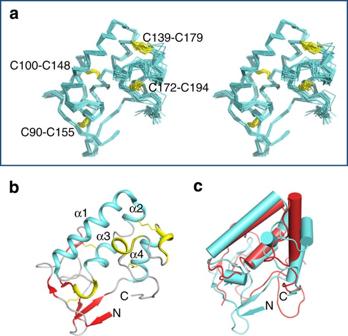Figure 3: Solution structure of the Smo CRD. (a) Stereo view of the backbone atoms (N, Cαand C′) of the 20 superimposed structures of Smo CRD with the lowest energy. The disulphides are indicated in yellow and are labelled for clarity. (b) Ribbon diagram of the Smo CRD showing the secondary structure elements. The structure with the lowest energy is used to describe the secondary structure elements. The colour scheme is as follows: cyan: alpha helices; red: β strands; yellow: 310helices; grey: random coil. (c) Superimposition of the Smo CRD with FzD CRD. The Smo CRD is represented in cyan and the FzD8 CRD is represented in red. The helices in both proteins are shown as cylinders and the beta-strands as arrowheads. All figures were generated using PyMol. Figure 3: Solution structure of the Smo CRD. ( a ) Stereo view of the backbone atoms (N, C α and C′) of the 20 superimposed structures of Smo CRD with the lowest energy. The disulphides are indicated in yellow and are labelled for clarity. ( b ) Ribbon diagram of the Smo CRD showing the secondary structure elements. The structure with the lowest energy is used to describe the secondary structure elements. The colour scheme is as follows: cyan: alpha helices; red: β strands; yellow: 3 10 helices; grey: random coil. ( c ) Superimposition of the Smo CRD with FzD CRD. The Smo CRD is represented in cyan and the FzD8 CRD is represented in red. The helices in both proteins are shown as cylinders and the beta-strands as arrowheads. All figures were generated using PyMol. Full size image Table 1 NMR and refinement statistics used for calculating the structure of Smo CRD . Full size table The cysteines in the Smo CRD Structure analysis shows that the eight conserved cysteines in Smo CRD form four disulphide bonds. The chemical shifts observed for the cysteine C-alpha and C-beta carbons are suggestive that all the cysteines are oxidized [29] . The disulphide bond pattern was determined based on the intermolecular nuclear Overhauser effects (NOEs) observed between the β-protons of the cysteine residues and is as follows: C90-C155, C100-C148, C139-C179 and C172-C194 ( Fig. 3a ). To study the structural and biological relevance of these disulphide bonds, we mutated the cysteines individually to alanine, and checked the ability of the cysteine to alanine Myc-Smo mutants to rescue Hh-induced reporter gene in a smo -knockdown background. C100A, C148A, C172A and C194A were able to rescue Hh-induced reporter gene induction to wild-type levels ( Fig. 2 ) indicating that the C100-C148 and C172-C194 disulphide bonds are not essential for a functional CRD. Conversely, C90A, C139A, C155A and C179A showed attenuated rescue of the Hh-induced reporter gene induction ( Fig. 2 ), suggesting that the C90-C155 and C139-C179 disulphide play critical roles in maintaining the integrity of the CRD structure. Indeed, additional indirect immunofluorescence revealed that Smo cysteine to alanine mutants that were compromised in their ability to signal were retained in the endoplasmic reticulum (ER), overlapping with the ER marker protein Calreticulin-GFP-KDEL ( Fig. 4a and Supplementary Fig. S1a ). ER retention is probably because of altered protein folding resulting from the loss of essential disulphide bridges. However, such misfolding did not trigger obvious degradation of Smo protein, as the cysteine to alanine mutants were present at protein levels similar to and greater than that of wild-type Smo ( Supplementary Fig. S1b , lane 2 compared with lanes 3–6). Although it is difficult to understand the cause of higher protein levels for cysteine to alanine mutants, we speculate that it may be due to the misfolded Smo mutants failing to exit the ER and cycle to the plasma membrane to be phosphorylated and desensitized like the wild-type protein [30] , [31] . 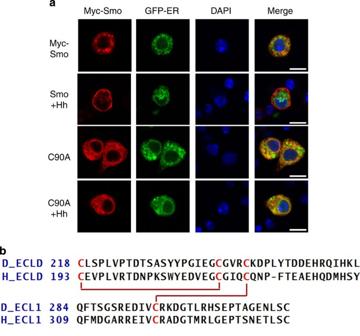Figure 4: Subcellular localization of the cysteines essential for Smo signalling. (a) CRD mutants with compromised signalling activity have altered subcellular localization. Cl8 cells expressing wild type or the indicated Myc-Smo-mutant protein, in the presence of Hh (+) or empty vector control, were examined by indirect immunofluorescence. Wild-type Smo translocates to the plasma membrane in response to Hh, whereas Smo CRD cysteine to alanine-mutant C90A that was required for maximal Hh reporter gene induction was largely retained in the ER. Smo was detected using anti-Myc (red), Calreticulin-GFP-KDEL marks the ER (green) and DAPI (blue) marks the nucleus. Scale bar, 10 μM. (b) Sequence alignment of theDrosophila(D) Smo ECLD and ECL1 with the human (H) Smo ECLD and ECL1. The cysteines engaged in disulphide bond formation in human Smo are conserved inDrosophila. The red lines indicate the disulphide bond pattern. Figure 4: Subcellular localization of the cysteines essential for Smo signalling. ( a ) CRD mutants with compromised signalling activity have altered subcellular localization. Cl8 cells expressing wild type or the indicated Myc-Smo-mutant protein, in the presence of Hh (+) or empty vector control, were examined by indirect immunofluorescence. Wild-type Smo translocates to the plasma membrane in response to Hh, whereas Smo CRD cysteine to alanine-mutant C90A that was required for maximal Hh reporter gene induction was largely retained in the ER. Smo was detected using anti-Myc (red), Calreticulin-GFP-KDEL marks the ER (green) and DAPI (blue) marks the nucleus. Scale bar, 10 μM. ( b ) Sequence alignment of the Drosophila (D) Smo ECLD and ECL1 with the human (H) Smo ECLD and ECL1. The cysteines engaged in disulphide bond formation in human Smo are conserved in Drosophila . The red lines indicate the disulphide bond pattern. Full size image The cysteines in the ECLD of Smo In addition to the cysteines of the CRD (V85-K202), the Drosophila Smo ECD has five other conserved cysteines, at positions 84, 203, 218, 238 and 242. In the three-dimensional (3D) structure of the Drosophila Smo CRD, the amino- and the carboxy termini are in close proximity ( Fig. 3b ), implying that C84 and C203 may form a disulphide bond. Nevertheless, mutation of C84 and C203 to alanine does not alter the ability of Smo to rescue reporter gene induction in the smo -knockdown background ( Fig. 2 ), suggesting that they are either not engaged in a disulphide bond or the disulphide bond is not crucial in defining the 3D fold of the CRD. However, when C218, C238 and C242 of the ECLD were mutated individually to alanine, they expressed at near-normal levels ( Supplementary Fig. S1c ), but failed to rescue Hh-induced reporter gene induction following endogenous smo knockdown ( Fig. 2 ). C218, C238 and C242 of Drosophila Smo are homologous to C193, C213 and C217 of human Smo ( Fig. 4b ). The crystal structure of the human Smo shows that the ECLD is stabilized towards the ECL by disulphide bonds between C193 and C213 of the ECLD and C217 of the ECLD and C295 ECL1 loop [14] ( Fig. 4b ). Hence, C218 and C238 in the ECLD of Drosophila Smo may form a disulphide bond and C242 in the ECLD is likely to form a disulphide bond with C320 in ECL1 of Drosophila Smo. Thus, cysteines both in the Smo CRD and ECD linker play an important role in maintaining the conformation of Smo essential for downstream signalling. Drosophila Smo CRD binds to the glucocorticoid Bud Smo activity can be modulated by small-molecule inhibitors such as cyclopamine, which binds in the orthosteric binding site located within a cavity in the 7TM bundle [14] , [24] . The FzD CRD binds to its endogenous ligand Wnt underscoring the ligand-binding capability of the CRDs [16] , [18] . Therefore, we decided to test whether the Drosophila CRD might bind to 20-OHC or Bud. Because of a solubility issue with 20-OHC, we carried out all experiments with Bud. We used NMR chemical shift perturbations (CSPs) to identify the residues that are involved in binding [32] , since this method allows us to determine precisely the amino-acid residues involved in the interaction [33] . Despite recent reports stating the inability of 20-OHC to bind to the Drosophila Smo protein, we tested whether Bud bound to Drosophila Smo CRD [25] . In the 2D 1 H– 15 N HSQC spectra of Smo CRD in the absence and presence of an increasing concentration of the ligand Bud, CSPs induced by the binding of Bud are clearly observed indicating Bud bound to the CRD ( Supplementary Figs S2a and S3 ). The normalized CSP for each residue of Smo in the presence of Bud is shown in Fig. 5a . The residues that have significant CSP are further shown in the backbone ‘ribbon’ representation of the Smo CRD, wherein the thickness of the ribbon is proportional to CSP values observed on binding of Bud to Smo CRD ( Fig. 5b ). The results show that the residues of Smo CRD that have the largest CSPs induced by the bound Bud are located between the first helix and the C-terminus 3 10 helical domain as it folds back between the first and second helix. As a control, we tested the ability of cyclopamine to bind and induce CSPs within the Smo CRD and Smo CRD did not bind to cyclopamine at a ratio of 1:2 of protein to ligand [24] ( Supplementary Fig. S2b ). 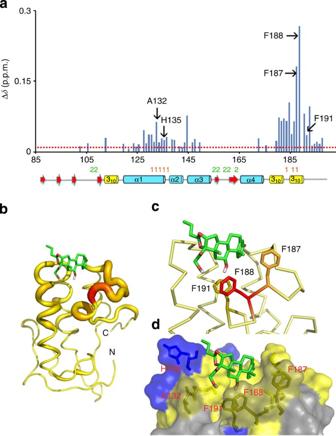Figure 5:DrosophilaSmo CRD binds to the glucocorticoid Bud. (a) CSPs of Smo CRD on addition of Bud are plotted versus residue numbers. The red line indicates CSP greater than 0.01 p.p.m. The residues labelled in black form the Bud-binding pocket on Smo CRD as analysed from the HADDOCK-docking experiments. The mouse FzD8–Wnt interacting ‘site 1’ and ‘site 2’ residues are shown in orange and green, respectively. The corresponding secondary structure elements of theDrosophilaSmo CRD are represented below the plot. (b) ‘Ribbon’ representation of the Smo CRD. The backbone thickness of the ribbon is directly proportional to the weighted sum (in p.p.m.) of the1H and15N chemical shifts on binding to the ligand Bud. (c,d) Results of the HADDOCK docking of Bud on Smo CRD. (c) The aromatic side chains of the Bud contacting Smo CRD residues are shown. (d) Surface representation of the residues that interact with Bud are shown in yellow and the positively charged H135 is shown in blue. Figure 5: Drosophila Smo CRD binds to the glucocorticoid Bud. ( a ) CSPs of Smo CRD on addition of Bud are plotted versus residue numbers. The red line indicates CSP greater than 0.01 p.p.m. The residues labelled in black form the Bud-binding pocket on Smo CRD as analysed from the HADDOCK-docking experiments. The mouse FzD8–Wnt interacting ‘site 1’ and ‘site 2’ residues are shown in orange and green, respectively. The corresponding secondary structure elements of the Drosophila Smo CRD are represented below the plot. ( b ) ‘Ribbon’ representation of the Smo CRD. The backbone thickness of the ribbon is directly proportional to the weighted sum (in p.p.m.) of the 1 H and 15 N chemical shifts on binding to the ligand Bud. ( c , d ) Results of the HADDOCK docking of Bud on Smo CRD. ( c ) The aromatic side chains of the Bud contacting Smo CRD residues are shown. ( d ) Surface representation of the residues that interact with Bud are shown in yellow and the positively charged H135 is shown in blue. Full size image On the basis of NMR studies, we generated the docked structure of Bud bound to Smo CRD using the program HADDOCK (High Ambiguity Driven protein–protein Docking) [34] . The CSP data on the Smo CRD and the bound Bud were used as ambiguous restraints ( Supplementary Table S1 ) for docking and generating 1,000 binding poses. The structure with the lowest binding energy was selected and this agrees with the CSP data on the Smo CRD ( Fig. 5b ). The modelled structure showed that Bud is buried into a hydrophobic surface formed by the residues A132, H135, F187, F188 and F191 on the Smo CRD ( Fig. 5c,d ). F191 is conserved in the vertebrate Smo family, whereas F188 is a tryptophan in vertebrate Smo ( Fig. 1 ). The conservation of these residues in the vertebrate family, and the recent demonstration that the domain engages 20-OHC [25] , [26] , suggests that this pocket may have an important role in binding an as yet unidentified allosteric regulator of Drosophila Smo. To determine whether Bud would attenuate signalling by the Drosophila Smo protein, we treated Cl8 cells with increasing concentrations of Bud, and observed an ∼ 20–40% reduction in Hh-induced reporter gene activity ( Supplementary Fig. S4 ). Thereby, we speculate that Bud acts as a weak, synthetic mimic of an endogenous ligand for the Drosophila Smo CRD, displacing it from this binding pocket. The human Smo CRD binds to the glucocorticoid Bud Recent reports indicate that 20-OHC binds the vertebrate Smo CRD [25] , [26] . We therefore tested the binding of Bud to human Smo CRD. The recombinant human Smo CRD (G65-G177) was expressed and purified using the E. coli expression system. Similar to the studies of Drosophila Smo CRD, 15 N- and 13 C-labelled protein was prepared in 10 mM deuterated acetic acid buffer and 10% D 2 O (volume/volume) at pH 5. In the 2D 1 H– 15 N HSQC spectra of human Smo CRD, all the amide resonances of the 113 residues were assigned except two residues, L73 and R74. NMR titration experiments were performed to determine the specific residues involved in ligand binding. The 2D 1 H– 15 N HSQC spectra of human Smo CRD in the absence and presence of an increasing concentration of Bud showed that Bud bound to human Smo CRD as well ( Supplementary Figs S5 and S6 ). The normalized CSP for each residue of human Smo CRD in the presence of Bud is shown in Fig. 6a . Comparing with Drosophila Smo CRD ( Fig. 5a ), Bud binds to human CRD in a similar manner. However, there are some clear differences. For example, a smaller number of residues in human Smo CRD had CSPs induced by the binding of Bud, and the absolute values of CSPs observed in human Smo CRD are smaller. Moreover, the binding affinities measured from different residues in human Smo CRD are clustered around 45 μM, whereas those obtained from residues in Drosophila Smo CRD range from 200 to 1,000 μM indicating that Bud binding induced backbone conformational stabilization in Drosophila CRD [35] . Nevertheless, judged by the NMR titration data, it seemed that Bud binds to human Smo CRD with higher affinity ( Supplementary Figs S3 and S6 ). Although NMR is a useful method for determining specific protein ligand interactions in solution, it is not the ideal method for calculating dissociation constants [36] . The associated systemic error in calculating K d values from NMR is probably caused by the averaging effect during NMR experiments [37] . K d values calculated by this method can only be treated as the upper limit for interaction. Therefore, we validated the binding affinity measurements using additional experiments. Indeed, using Bio-layer interferometry (BLI), we found that Bud bound to Drosophila Smo CRD with a K d value of 120±98 μM and bound to human Smo CRD with a K d value of 52±16 μM ( Fig. 6b,c ). Both NMR and BLI data suggest that Bud binds to human Smo CRD better than Drosophila Smo CRD. 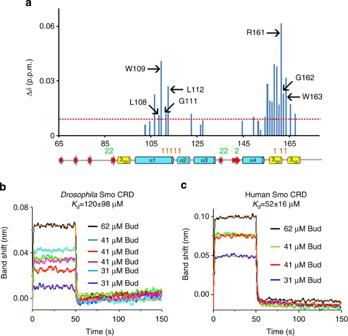Figure 6: Analysis of the binding of Bud to human Smo CRD. (a) CSPs of human Smo CRD on addition of Bud are plotted versus residue numbers. Dotted red line indicates CSP greater than 0.01 p.p.m. L108, W109, G111, L112 and R161 are homologous to the mouse Smo residues that interact with 20-OHC. G162 is homologous toDrosophilaF187 and W163 is homologous toDrosophilaSmo F188 that interacts with Bud. All these residues map to the ‘site 1’ of mouse FzD8–Wnt interaction. ‘Site 1’ and ‘site 2’ residues of mouse FzD8–Wnt interaction are shown in orange and green, respectively. The secondary structure elements as inDrosophilaSmo CRD structure are shown below the plot. (b) BLI-binding assays show that Bud binds toDrosophilaSmo CRD. The SSA sensors with biotinylatedDrosophilaSmo CRD were exposed to three different concentrations of Bud (62, 41 and 31 μM). The processed data were fitted locally with the integrated fitting function by a 1:1 binding model (orange line). The respectiveKdvalues obtained by curve fitting were 89 μM (62 μM Bud, black line), 74 μM (41 μM Bud, green line), 59 μM (41 μM Bud, red line), 318 μM (41 μM Bud, magenta line), 93 μM (31 μM Bud, cyan line) and 85 μM (31 μM Bud, blue line). The averageKdvalue ofDrosophilaSmo CRD for Bud was 120±98 μM. (c) BLI-binding assays show that Bud binds to human Smo CRD. The experimental and data analysis procedure were same as described above. The respectiveKdvalues obtained by curve fitting were 74 μM (62 μM Bud, black line), 37 μM (41 μM Bud, green line), 44 μM (41 μM Bud, red line) and 54 μM (31 μM Bud, blue line). The averageKdvalue of human Smo CRD for Bud was 52±16 μM. Figure 6: Analysis of the binding of Bud to human Smo CRD. ( a ) CSPs of human Smo CRD on addition of Bud are plotted versus residue numbers. Dotted red line indicates CSP greater than 0.01 p.p.m. L108, W109, G111, L112 and R161 are homologous to the mouse Smo residues that interact with 20-OHC. G162 is homologous to Drosophila F187 and W163 is homologous to Drosophila Smo F188 that interacts with Bud. All these residues map to the ‘site 1’ of mouse FzD8–Wnt interaction. ‘Site 1’ and ‘site 2’ residues of mouse FzD8–Wnt interaction are shown in orange and green, respectively. The secondary structure elements as in Drosophila Smo CRD structure are shown below the plot. ( b ) BLI-binding assays show that Bud binds to Drosophila Smo CRD. The SSA sensors with biotinylated Drosophila Smo CRD were exposed to three different concentrations of Bud (62, 41 and 31 μM). The processed data were fitted locally with the integrated fitting function by a 1:1 binding model (orange line). The respective K d values obtained by curve fitting were 89 μM (62 μM Bud, black line), 74 μM (41 μM Bud, green line), 59 μM (41 μM Bud, red line), 318 μM (41 μM Bud, magenta line), 93 μM (31 μM Bud, cyan line) and 85 μM (31 μM Bud, blue line). The average K d value of Drosophila Smo CRD for Bud was 120±98 μM. ( c ) BLI-binding assays show that Bud binds to human Smo CRD. The experimental and data analysis procedure were same as described above. The respective K d values obtained by curve fitting were 74 μM (62 μM Bud, black line), 37 μM (41 μM Bud, green line), 44 μM (41 μM Bud, red line) and 54 μM (31 μM Bud, blue line). The average K d value of human Smo CRD for Bud was 52±16 μM. Full size image Classical GPCR signalling involves binding of ligands to the extracellular regions of the receptor, which induces a conformational change in the core of the 7TM domains to modulate signalling events in the cytoplasm [38] , [39] . Several studies have reported that GPCRs are regulated by natural ligands, as well as exogenous small molecules [38] , [39] , [40] , [41] . Furthermore, GPCRs have been reported to possess allosteric binding sites distinct from their orthosteric sites, which when bound by small-molecule modulators, induce distinct signal outputs [42] , [43] . In the FzD GPCR, the CRD functions to bind to the endogenous ligand Wnt, which interacts with the CRD at two sites [16] , [18] . The palmitate modification on Wnt engages a groove on the FzD8 CRD termed site 1, whereas the second Wnt-binding site on FzD8 CRD (site 2) is located on the opposite end and involves protein–protein interactions [18] . In the current studies, we showed that Bud interacts with Smo CRD residues analogous to site 1. Within the site 1 of human Smo R161 demonstrated the highest observed CSP. L108, W109, G111, L112, G162 and W163 also demonstrated CSPs. Consistent with these findings, a recent report shows that mutating the homologous murine Smo CRD residues ‘WGL’ (W113, G115 and L116) and R165 to alanine blocked the specific binding of 20-OHC to the Smo CRD and attenuated its signalling ability [26] . Furthermore, mutating murine L112 (human L108) and W113 (human W109) to equivalent Drosophila Smo CRD residues blocked 20-OHC binding [25] , suggesting that the site 1 is involved in the binding of hydroxyl-sterols and glucocorticoids. Drosophila Smo protein does not bind to 20-OHC in vitro [25] ; however, that does not preclude the fact that there could be an as yet unidentified endogenous ligand for Drosophila Smo CRD binding to this pocket. Consistent with this hypothesis, genetic experiments suggest that phospholipids could serve as the physiological molecules regulating Drosophila Smo activity [44] . The cache of identified Smo modulators dock on distinct sites on Smo to regulate signalling [14] , [24] , [45] , [46] . The extracellular region of Smo may be flexible ( Fig. 7a ). Small molecules may bind in the cavity of the 7TM domains ( Fig. 7b , right) and modulate signalling irrespective of CRD binding [14] , [24] . In the present study, we provide structural evidence identifying the specific residues in the Smo CRD that interact with the small-molecule modulator Bud. We speculate that these same residues bind the endogenous allosteric activator, and that activator binding to the CRD may cause a conformational shift that bridges the ECDs and the 7TM domains ( Fig. 7b , middle), similar to what is observed for class B GPCRs [40] , [41] , [47] . These shifts may enhance communication between the CRD and the 7TM domains to trigger structural alterations in the core and the cytoplasmic domains to regulate downstream signalling ( Fig. 7 ). 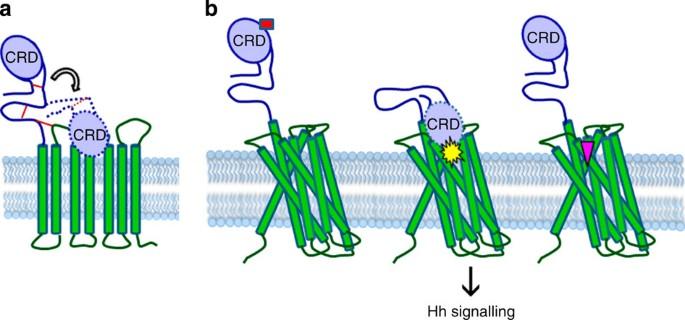Figure 7: A novel model for Smo allosteric regulation. (a) Smo CRD may be flexible. The disulphide bonds stabilizing Smo extracellular linker and ECL are shown in red lines. (b) Smo has more than one binding site. We propose that molecules like Bud bind to the Smo CRD (left, red rectangle) to alter its conformation and attenuate its signalling activity. Cyclopamine and vismodegib are known to bind near the orthosteric-binding site located in the cavity of the Smo 7TM domains (right, pink inverted triangle). We speculate that there is the possibility of a class of molecules (middle, yellow star), which would bind to the CRD and cause a conformational change of the Smo extracellular structures to bring it closer to the 7TM domains. This in turn might change the conformation of the transmembrane domains to regulate signalling. Figure 7: A novel model for Smo allosteric regulation. ( a ) Smo CRD may be flexible. The disulphide bonds stabilizing Smo extracellular linker and ECL are shown in red lines. ( b ) Smo has more than one binding site. We propose that molecules like Bud bind to the Smo CRD (left, red rectangle) to alter its conformation and attenuate its signalling activity. Cyclopamine and vismodegib are known to bind near the orthosteric-binding site located in the cavity of the Smo 7TM domains (right, pink inverted triangle). We speculate that there is the possibility of a class of molecules (middle, yellow star), which would bind to the CRD and cause a conformational change of the Smo extracellular structures to bring it closer to the 7TM domains. This in turn might change the conformation of the transmembrane domains to regulate signalling. Full size image Currently, the only Food and Drug Administration-approved therapeutic aimed at targeting Smo is the antagonist Vismodegib, which is likely to bind in the cavity of the 7TM domains and also make contacts with the ECLD and ECL [14] , [24] , [48] , [49] . Despite initial clinical success, resistance to this compound has been observed [48] . Thus, the need exists for developing second-generation drugs that can overcome the acquired drug resistance. On the basis of our data, we speculate that the Bud binding cleft in the Smo CRD could be evaluated for the development of novel antagonists of Smo. Bud is a clinically approved anti-inflammatory glucocorticoid steroid and has the advantage of acting on wild-type as well as Vismodegib-resistant Smo [23] , [50] . Thus, future investigation and identification of Bud-like molecules that bind to the Smo CRD with high affinity may represent a novel class of Smo regulators. Vector construction The Drosophila Smo CRD (V85-K202) was amplified from pET-SmoN 3 . The forward and the reverse primers used were 5′-ATA TAT CAT ATG GTC CGA CGT GCC CGT TGC-3′ and 5′-ATA TAC TCG AGT TAT TTC GTC GGA AAG AGT G-3′. The PCR-amplified product was cloned in pET-28a (+) and validated by nucleotide sequencing. To generate cysteine to alanine mutants, Smo-mutant expression vectors pAc-myc-smo [51] was mutated using QuickChange II Site Directed Mutagenesis Kit (Stratagene) using primers generated per manufacturer’s instructions. All mutations were verified by sequencing. Smo 5′-UTR double-stranded RNA (dsRNA) was generated using the Megascript T7 kit (Life Technologies) [15] . The human Smo CRD (G65-G177) was amplified from the smo complementary DNA purchased from Origene. The forward and the reverse primers used were 5′-TAT ATC ATA TGG GCC GGG CTG CCC CCT GC-3′ and 5′-ATA TAT CTC GAG TTA GCC TTC AGG GAA GCG-3′, respectively. The PCR-amplified product was cloned in pET-28a (+) and validated by nucleotide sequencing. Protein expression and purification For the expression of both the Drosophila and human-recombinant protein pET-28a-smoCRD was transformed into BL21 (DE3) cells. The cells were grown in 3-( N -morpholino) propane sulphonic acid minimal media supplemented with 15 N ammonium chloride and 13 C glucose as the sole source of nitrogen and carbon, respectively. Cells were grown to an optical density (OD 600 ) of 0.6 and induced with 1 mM isopropyl β- D -1-thiogalactopyranoside. The protein of interest accumulated in the inclusion bodies and was refolded from the same by the method of rapid dilution. The protein was further purified by reverse-phase HPLC using a C18 column (Hitachi) and gel filtration (AKTA) on a Hiload 16/60 Superdex 200 preparative grade column (GE Healthcare). NMR spectroscopy A 200-μM pure monomeric sample of the recombinant Drosophila (V85-K202) or human (G65-G177) Smo CRD was prepared in 10 mM deuterated acetic acid buffer and 10% D 2 O (volume/volume) for NMR experiments. All spectra were recorded using either 1 H, 15 N-labelled or 1 H-, 15 N- and 13 C-labelled protein on Bruker Avance 600 MHz or 800 MHz NMR spectrometers equipped with 1 H/ 15 N/ 13 C detect, triple resonance cryogenic inverse (TCI) probes at 25 °C. All spectra were processed using Topspin 3.0 NMR software (Bruker Biospin) and analysed using the program, CARA (computer aided resonance assignment) [52] . The backbone chemical shift assignment were obtained using the standard triple-resonance assignment strategy using the 2D 1 H– 15 N HSQC and 3D HNCA, HNCACB, CBCA(CO)NH, HN(CA)CO and HNCO NMR experiments. The aliphatic side-chain resonance assignments were obtained using HBHA(CBCACO)NH and (H)CCH-total correlation spectroscopy. Distance constraints for the structure calculation were derived from 15 N; 13 C resolved 1 H– 1 H NOESY with a mixing time of 100 ms. CSP experiments were carried out using 15 N-labelled Drosophila or human Smo CRD. 1 H– 15 N HSQC spectra were recorded in the absence and presence of an increasing concentration of Bud. K d values were calculated by a nonlinear least-squares analysis in the program Origin using the equation (1) where [L] is the concentration of the ligand, [P] is the concentration of the protein, Δ δ is the observed chemical shift change and Δ δ max is the normalized chemical shift change at saturation, calculated using equation (2) where Δ δ is the chemical shift in p.p.m. A stock solution of 50 mM Bud (Sigma) was made in deuterated dimethylsulphoxide (DMSO) for use in NMR titration experiments. The concentration of DMSO in the NMR titration experiment was maintained at or below 1%. A control experiment was done by titrating 1% DMSO and no CSPs were observed. Structure calculation and refinement An automated program UNIO [53] was used for the NOE assignment and all these assignments were manually checked. Integrated NOE peaks were calibrated and converted to distance constraints with the program CALIBA [54] . A total of 1,421 meaningful distance constraints were derived from the NMR data and used as input for structure calculation using the program CYANA 2.1 (ref. 54 ). The structure was refined using 139 dihedral angle constraints and 22 hydrogen bond constraints. The dihedral angles were generated by the program TALOS+ (ref. 55 ), which uses six kinds (HN, HA, CA, CB, CO and N) of chemical shift values for a given residue as input to give the phi, psi angles. The Ramachandran statistics are as follows: most favourable 72.5%, additionally allowed 25.7%, generously allowed 1.6% and disallowed 0.2%. Also, four disulphide bonds were added as additional constraints between residues, C90-C155, C100-C148, C139-C179 and C172-C194. A total of 100 conformers were initially generated and 20 conformers with the lowest target function were used to represent the 3D NMR structure. Structural modelling of Smo CRD in complex with Bud To calculate the structure of the CRD–Bud complex, we used the simulated annealing protocol in the program CNS [34] . All calculations were done using the program HADDOCK 2.1 (ref. 34 ). Topology and parameter files for Bud were generated by using xplo2d, and the charge parameters of Bud were calculated by using the antechamber module in the AMBER10 software package [56] . We used ambiguous distance restraints resulting from the CSPs of 1 H– 15 N Smo CRD ( Supplementary Table S1 ). To define the active and passive residues, we also calculated a relative accessible surface area by NACCESS [57] . One thousand initial structures of the Smo CRD–Bud complex were generated and the final 10 structures of the complex with the lowest energy were selected manually that were consistent with the CSPs on Smo CRD following Bud binding. Lysate preparation and functional assays Expression vectors and dsRNA were transfected using Lipofectamine 2000 according to the manufacturer’s instructions. For rescue reporter experiments, ∼ 1.5 × 10 6 Cl8 cells were co-transfected with 500 ng Smo 5′-UTR dsRNA, 100 ng ptcΔ136-luciferase [27] 10 ng pAc-Renilla [51] and, unless otherwise indicated, 100 ng of pAc-Hh (+Hh) and 50 ng of the indicated pAc-myc-smo expression vector. DNA and RNA content were normalized with control dsRNA and/or pAc5.1A . Forty-eight hours post transfection, cells were lysed and luciferase activity measured using the Dual Luciferase Assay System (Promega) [15] . For all reporter assays, experiments were performed a minimum of two times in duplicate or triplicate and all data were pooled. Error bars indicate s.e.m. For the Bud treatment, Cl8 cells were treated with the indicated concentration of Bud (Sigma) or DMSO vehicle. Bud was added in serum-free M3 media (Sigma) 24 h post transfection. Cells were treated with Bud for 24 h before measuring luciferase activity. Experiments were performed at least three times in duplicate and all data were pooled. For biochemical analysis, ∼ 6 × 10 6 Cl8 cells were transfected with 5 μg of the indicated pAc-myc-smo expression vector and 3 μg of pAc-Hh , as indicated. DNA content was normalized with empty pAc5.1A . Forty-eight hours post transfection, cells were lysed in NP-40 lysis buffer (1% NP-40, 150 mM NaCl, 50 mM Tris, 50 mM NaF, 0.5 mM dithiothreitol and 1 × protease inhibitor cocktail (Roche), pH 8.0), and centrifuged for 10 min at 2,000 × g . The resulting supernatants were analysed by SDS–polyacrylamide gel electrophoresis and western blot using anti-Myc (Roche, catalogue number 11667149001 diluted 1:5,000) and anti-Kinesin (Cytoskeleton, AKIN01-A, diluted 1:10,000). Full scans of the western blots are represented in Supplementary Fig. S7 . Antibodies were diluted in Tris-buffered saline with 0.1% Tween and 5% powdered milk. Immunofluorescence and microscopy For immunofluorescence experiments, ∼ 6 × 10 6 Cl8 cells were transfected with 2 μg of Calreticulin-GFP-KDEL [58] , 2 μg pAc-Hh and 2 μg of the indicated pAc-myc-smo expression vector. DNA content was normalized with pAc5.1A . Forty-eight hours post transfection, cells were re-plated on chamber slides, fixed using 4% formaldehyde and immunostained using anti-Myc (Roche, catalogue number 11667149001) [15] , Calreticulin-GFP-KDEL was used to mark the ER, and DAPI was used to mark the nucleus. Confocal images were collected using a Zeiss LSM 510 NLO Meta microscope. BLI assay The Octet RED instrument (FortéBio) was used to measure the interaction of Drosophila Smo CRD (or human Smo CRD) and Bud. Super streptavidin (SSA) sensors were used to catch the biotinylated target protein. Biotinylation of the target protein was achieved by incubating 200 μl of 1.0 mg ml −1 EZ-Link NHS-LC-Biotin (Thermo Scientific) with 100 μl of 0.2 mM target protein in 0.1 M potassium phosphate buffer, pH 6.5 for 15 h on a rocking platform at room temperature. Excess unreacted biotin was removed by three successive dialysis under the same buffer conditions. Before the start of the assay, the SSA sensors were pre-wet in 0.1 M potassium phosphate buffer, pH 6.5 with 0.01% Trion-X100 for 10 min. For the binding affinity assay, 3 ∼ 5 μM biotinylated protein was immobilized on the SSA sensor by incubating for 30 min. Subsequently, the free streptavidin sites were quenched by incubating with 0.5 mM biocytin (Thermo Scientific) for 10 min. Excess protein and biocytin were removed by washing with 0.1 M potassium phosphate, pH 6.5 for 10 min. To determine the binding affinity of Drosophila Smo CRD (or human Smo CRD) to Bud, three different concentrations of Bud (62, 41 and 31 μM) were used. The association step for 50 s was followed by the dissociation step for 100 s. The assay buffer used was 0.1 M potassium phosphate, pH 6.5 with 0.5% DMSO. Biocytin-loaded SSA sensor without loading biotinylated protein was used as a control to correct the systematic optical artefacts and baseline drifts. All steps were performed at 30 °C with 1,000 r.p.m. rotary shaking. The processed data were fitted locally with the integrated fitting function using the 1:1 binding model in FortéBio analysis software (v6.4). The kinetic constants k on (on-rate constant), k off (off-rate constant) and K d were calculated from curve fitting. How to cite this article: Rana, R. et al. Structural insights into the role of the Smoothened cysteine-rich domain in Hedgehog signalling. Nat. Commun. 4:2965 doi: 10.1038/ncomms3965 (2013).